Tertiary structural elements determine the extent and specificity of messenger RNA editing The specificity and extent of RNA editing by ADAR enzymes is determined largely by local primary sequence and secondary structural imperfections in duplex RNA. Here we surgically alter conserved cis elements associated with a cluster of ADAR modification sites within the endogenous Drosophila paralytic transcript. In addition to the local requirement for a central imperfect RNA duplex containing the modified adenosines, we demonstrate that a secondary RNA duplex containing splicing signals strongly modulates RNA editing. A subtle non-coding mutation, extending base pairing of this accessory helix, confers significant phenotypic consequences via effects on splicing. Through mutation/counter-mutation, we also uncover and functionally replace a highly conserved intronic long-range tertiary pseudoknot that is absolutely required for deamination of one particular adenosine in the central duplex. Our results demonstrate that complex RNA tertiary structures, which may be difficult to predict computationally, form in vivo and can regulate RNA-editing events. The spatial folding of RNA in vivo poses an experimentally difficult but vital issue for key biological processes. Recognition of double-stranded RNA substrates by proteins depends largely on target structure [1] . Such proteins bind through structural motifs seeking generic dsRNA features rather than primary nucleotide sequence. Although recent evidence suggests that dsRNA-binding domains (RBDs) are capable of primary sequence recognition via the shallow minor groove of duplex RNA [2] , three-dimensional RNA structure has a major role in highly specific protein-RNA recognition, supporting diverse cellular functions such as splicing, RNA interference and translation. ADAR ( a denosine d e a minases that act on R NA) family members possess dsRBDs, recognize diverse RNA substrates and catalyse the deamination of adenosines into inosines in a post-transcriptional process known as A-to-I RNA editing [3] . As the chemical properties of inosine mimic those of guanosine, cellular machines, including the ribosome, interpret inosine as guanosine. Therefore, RNA editing effectively causes an adenosine to guanosine change in the primary sequence of mRNAs, potentially recoding the resulting peptides. A-to-I editing is thought to exist as a mechanism to expand protein repertoires within the nervous system [4] , [5] , [6] . ADARs are strikingly conserved among metazoa [3] , [7] and engineered model organisms lacking ADAR activity display severe neurological phenotypes, including seizures and neurodegeneration [8] , [9] , [10] , [11] . Furthermore, ADARs are localized to the neuronal nucleus [12] and nucleolus [13] , supporting the role of editing in nascent, immature RNA molecules. One exemplar Drosophila neuronal editing substrate is paralytic ( para ), an essential action potential sodium channel gene in the fly genome [14] . In contrast, nine voltage-gated sodium channel genes (Na v 1.1-Na v 1.9) are encoded in the mammalian genome [15] . Yet para transcripts are extensively alternatively spliced and edited ( Fig. 1a ), post-transcriptional modifications that result in over 2 million potential sodium channel isoforms [16] . 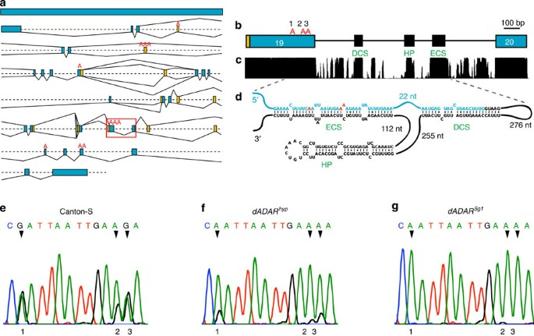Figure 1: Organization of para exon 19 editing sites and ADAR dependence. (a) Theparalocus contains 26 constitutive exons (blue), 13 alternative exons (yellow) and 11 sites of RNA editing (red). The boxed region in (a) is enlarged in (b), showing the three nearby editing sites in constitutive exon 19. (c) Sequence conservation of the region in (b) from 13 species ofDrosophilidaefound in the UCSC Genome Browser. Three regions of intronic homology, the ECS (‘editing site complementary sequence’), DCS (‘donor-site complementary sequence’), and HP are putativecissequences. (d) The indicated region of theparatranscript from exon 19 (blue) and the downstream intron (black), folded in Sfold, show the conservedcissequences denoted in (c) involved in double-stranded structures. Edited adenosines are shown in red. (e) Wild-type (Canton-S) editing at the three sites in exon 19 is apparent as mixed A/G peaks in electropherograms from reverse-transcribedparamRNA. (f) Editing at these sites is sensitive to dADAR levels, as editing in a hypomorphicdADARmutant (dADARhyp) are greatly reduced. (g) Editing is completely abolished in thedADAR5g1null mutant. Figure 1: Organization of para exon 19 editing sites and ADAR dependence. ( a ) The para locus contains 26 constitutive exons (blue), 13 alternative exons (yellow) and 11 sites of RNA editing (red). The boxed region in ( a ) is enlarged in ( b ), showing the three nearby editing sites in constitutive exon 19. ( c ) Sequence conservation of the region in ( b ) from 13 species of Drosophilidae found in the UCSC Genome Browser. Three regions of intronic homology, the ECS (‘editing site complementary sequence’), DCS (‘donor-site complementary sequence’), and HP are putative cis sequences. ( d ) The indicated region of the para transcript from exon 19 (blue) and the downstream intron (black), folded in Sfold, show the conserved cis sequences denoted in ( c ) involved in double-stranded structures. Edited adenosines are shown in red. ( e ) Wild-type (Canton-S) editing at the three sites in exon 19 is apparent as mixed A/G peaks in electropherograms from reverse-transcribed para mRNA. ( f ) Editing at these sites is sensitive to dADAR levels, as editing in a hypomorphic dADAR mutant ( dADAR hyp ) are greatly reduced. ( g ) Editing is completely abolished in the dADAR 5g1 null mutant. Full size image ADAR proteins contain at least one dsRBD, congruent with edited adenosines residing within dsRNA structures [17] . Nevertheless, very few ADAR targets have been probed to reveal the extent to which three-dimensional properties contribute to editing specificity. Complicating this picture is the observation that the isolated ADAR catalytic domain, lacking dsRBDs, edits certain target dsRNAs [18] , and that mutations in the catalytic domain of human ADAR2 cause altered editing site specificity [19] . At the RNA level, ADAR substrates range from perfectly complementary long RNA hairpins (HPs), which are promiscuously hyper-edited at up to 40% of adenosines [20] , to shorter (~25 bp) imperfectly paired substrates, which are specifically edited at one or a few adenosines [21] . The menagerie of specifically edited substrates includes simple short HPs, such as the 71-nt stem-loop directing editing at the mammalian GluR-2 R/G site [22] , as well as comparatively enormous pseudoknotted structures, such as that found in the Drosophila synaptotagmin-1 transcript, whose elements span thousands of nucleotides [23] . Most RNA structures that recruit ADAR proteins involve exonic editing sites that interact via base pairing with complementary conserved intronic cis sequences. The diversity of ADAR targets provides a unique source for studying RNA–protein and RNA–RNA interactions. Containing 11 highly specific editing sites ( Fig. 1a ), paralytic mRNA provides an exceptional opportunity to study enzyme–substrate interactions directing RNA editing. However, previous in vivo studies of paralytic have only demonstrated an implied necessity for secondary structure [24] . Here we describe the in vivo molecular consequences of RNA structural perturbations, introduced via knock-in into the endogenous para locus, using homologous recombination (HR) [25] . These mutations probe conserved cis sequences in predicted RNA structures and establish the necessity of imperfect double-strandedness around editing sites. We also reveal the presence of an accessory duplex formed around the splicing-donor site, which may mediate an interaction between RNA splicing and the extent of editing. Finally, our data demonstrate that a highly conserved tertiary pseudoknot (PK) is indispensable in directing ADAR to only one of three nearby adenosines. Replacing the PK with a functional analogue indicates the generality of the mechanism. Our data demonstrate that proximity of editing sites within a central duplex does not imply functional coupling. We show that extent and selectivity of editing can be determined by structural components assembled from distant sequence elements. RNA structural predictions for RNA-editing sites The Drosophila paralytic transcript possesses three nearby edited adenosines (1–3) in exon 19 ( Fig. 1b ), apparent as mixed A/G peaks in wild-type electropherograms of RT–PCR products ( Fig. 1e ), and is predicted to form a dsRNA secondary structure ( Fig. 1d ). Editing is sensitive to levels of Drosophila ADAR (dADAR), as flies carrying a hypomorphic dADAR allele (~80% dADAR reduction) [26] show reduced editing levels ( Fig. 1f ) and dADAR null males [9] do not edit these sites ( Fig. 1g ). Editing at these three adenosines is conserved across Drosophila species [24] ( Supplementary Fig. S1 ). Previous study of these sites predicted and experimentally validated the minimal sequences necessary for RNA editing [24] . However, only two species were compared when making these predictions. A more comprehensive study could reveal additional conserved elements. Therefore, we obtained sequences from 37 species of the genus Drosophilidae ( Supplementary Fig. S2 ). Sequence alignments revealed several areas of extreme intron conservation ( Fig. 1c , Supplementary Fig. S2 ). The RNA folding algorithm Sfold [27] predicted structural features of the paralytic transcript in this region, including three striking features corresponding to regions of high sequence conservation ( Fig. 1c,d ). The expected central duplex places the three editing sites within a 77 bp-long imperfect duplex formed between the exon and downstream intron possessing homology to the edited region (‘editing site complementary sequence,’ ECS; Supplementary Fig. S3a ). In addition, a highly invariant area of the intron, the ‘donor-site complementary sequence’ (DCS; Supplementary Fig. S3b ), is predicted to form a secondary RNA duplex encompassing the 5′-splice donor site. Finally, a predicted intronic local HP of unknown function is highly conserved in all species surveyed ( Supplementary Fig. S3c ). A central RNA duplex is required for RNA editing in vivo Traditional experimental manipulation of RNA-editing structures are usually conducted in vitro [28] or with mini-gene reporters in culture [29] , [30] . Many of these studies generally recapitulate editing and delineate important cis elements. We chose to use ends-out HR to study the in vivo details of RNA editing, because precise mutation of genes preserves endogenous gene regulation. [31] Briefly, the process of HR introduces mutations into the genome, as well as a 76-bp LoxP remnant directed to a region of the intron with low-sequence conservation [31] ( Fig. 2a ). The targeting construct encompasses a mini-white marker gene flanked by LoxP sites and two homology arms into which the desired mutations are engineered ( Fig. 2b ). After targeting, Cre-recombinase removes the mini-white gene, leaving a single LoxP remnant. A wild-type construct containing no mutations in the para locus provides the appropriate control for all other mutants ( Figs 2c , 3a and 5a). 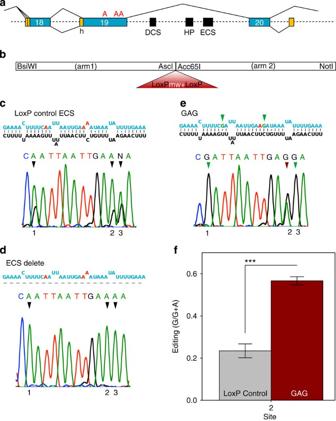Figure 2: Editing mutations introduced by HR demonstrate necessity of central duplex. (a) The region of theparalocus targeted by HR encompasses exon 19 and the putativeciselements (black). (b) The targeting construct for HR involves two ‘arms’ (white), homologous to the endogenousparalocus and bordered by unique restriction sites. Amini-whitereporter gene flanked by LoxP sites (red) is situated between the arms and targeted to a region in the intron of low sequence conservation. (c) As a proper control, a construct containing wild-type arms is targeted to create the LoxP control line, which is wild-type except for the LoxP remnant in the intron. Editing at the three sites occurs in this control. (d) When the 39 nt ECS introniccissequence is deleted through HR (‘ECS delete’), editing is completely abolished at all three adenosines. (e) The ‘GAG’ mutation replaces the non-silent first (Glu>Arg) and third (Asn>Asp) adenosines with guanosines (green carrots), resulting in sodium channel peptides representing only the completely edited form. (f) The GAG mutation (red) causes editing at the silent site 2 to increase compared with the LoxP control (grey). Bars represent 95% confidence intervals from three biological replicates (***P<0.0001, one-way ANOVAs with Dunnettpost-hoctests (α=0.05), please seeSupplementary Fig. S10afor raw data and specificP-values). Figure 2: Editing mutations introduced by HR demonstrate necessity of central duplex. ( a ) The region of the para locus targeted by HR encompasses exon 19 and the putative cis elements (black). ( b ) The targeting construct for HR involves two ‘arms’ (white), homologous to the endogenous para locus and bordered by unique restriction sites. A mini-white reporter gene flanked by LoxP sites (red) is situated between the arms and targeted to a region in the intron of low sequence conservation. ( c ) As a proper control, a construct containing wild-type arms is targeted to create the LoxP control line, which is wild-type except for the LoxP remnant in the intron. Editing at the three sites occurs in this control. ( d ) When the 39 nt ECS intronic cis sequence is deleted through HR (‘ECS delete’), editing is completely abolished at all three adenosines. ( e ) The ‘GAG’ mutation replaces the non-silent first (Glu>Arg) and third (Asn>Asp) adenosines with guanosines (green carrots), resulting in sodium channel peptides representing only the completely edited form. ( f ) The GAG mutation (red) causes editing at the silent site 2 to increase compared with the LoxP control (grey). Bars represent 95% confidence intervals from three biological replicates (*** P <0.0001, one-way ANOVAs with Dunnett post-hoc tests ( α =0.05), please see Supplementary Fig. S10a for raw data and specific P- values). 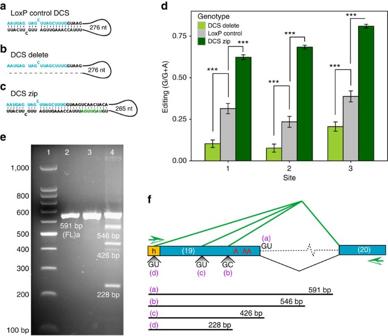Figure 3: Mutations in the donor-site complementary sequence (DCS) affect editing and splicing. (a) In the LoxP control, the wild-type DCS intronic sequence is predicted to involve the donor site in secondary structure. (b) The ‘DCS delete’ mutation excises the conserved 24 nt DCScissequence from the intron. (c) Seven intronic nucleotides (green) are added to the wild-type DCS (‘DCS zip’), and are predicted to result in a more stable secondary structure around the splice donor. (d) Editing at all three sites significantly decreases in the ‘DCS delete’Drosophilalines compared with the LoxP control (grey), whereas editing significantly increases in animals homozygous for the ‘DCS zip’ allele. Bars represent 95% confidence intervals from three biological replicates (***P<0.0001, one-way ANOVAs with Dunnettpost-hoctests (α=0.05), please seeSupplementary Fig. S10afor raw data and specificP-values). (e) PCR was performed on cDNA reverse-transcribed fromparamRNA. Not allparatranscripts from the ‘DCS zip’ allele are full-length (FL). Lane 1, 100 bp ladder; lane 2, LoxP control; lane 3, DCS delete; lane 4, DCS zip. Sizes of bands are indicated on the 1.5% agarose gel. (f) Aberrant bands from (e) were isolated and sequenced to determine the activated cryptic donor sites within constitutive exon 19 (blue) and alternative exon h (yellow). Primers (green) in exons h and 20 produce the full-length PCR product (a) from the wild-type splice donor. Aberrant shorter products (b–d) are formed owing to activation of cryptic alternative donor sites in exons h and 19. Full size image Figure 3: Mutations in the donor-site complementary sequence (DCS) affect editing and splicing. ( a ) In the LoxP control, the wild-type DCS intronic sequence is predicted to involve the donor site in secondary structure. ( b ) The ‘DCS delete’ mutation excises the conserved 24 nt DCS cis sequence from the intron. ( c ) Seven intronic nucleotides (green) are added to the wild-type DCS (‘DCS zip’), and are predicted to result in a more stable secondary structure around the splice donor. ( d ) Editing at all three sites significantly decreases in the ‘DCS delete’ Drosophila lines compared with the LoxP control (grey), whereas editing significantly increases in animals homozygous for the ‘DCS zip’ allele. Bars represent 95% confidence intervals from three biological replicates (*** P <0.0001, one-way ANOVAs with Dunnett post-hoc tests ( α =0.05), please see Supplementary Fig. S10a for raw data and specific P -values). ( e ) PCR was performed on cDNA reverse-transcribed from para mRNA. Not all para transcripts from the ‘DCS zip’ allele are full-length (FL). Lane 1, 100 bp ladder; lane 2, LoxP control; lane 3, DCS delete; lane 4, DCS zip. Sizes of bands are indicated on the 1.5% agarose gel. ( f ) Aberrant bands from ( e ) were isolated and sequenced to determine the activated cryptic donor sites within constitutive exon 19 (blue) and alternative exon h (yellow). Primers (green) in exons h and 20 produce the full-length PCR product (a) from the wild-type splice donor. Aberrant shorter products (b–d) are formed owing to activation of cryptic alternative donor sites in exons h and 19. Full size image We first assessed the role of the predicted ECS by deleting the 39 intronic nucleotides predicted to pair with the edited region. As expected, when the para ECS is deleted, editing is completely abolished ( Fig. 2d ) compared with the LoxP control ( Fig. 2c ). Although all three edited adenosines require the ECS-directed central duplex, editing at only the first and third sites alter amino acids (Glu to Arg, Asn to Asp, respectively). We next mutated the first and third edited adenosines to guanosines, mimicking complete ADAR modification at these sites ( Fig. 2e ). This mutation (‘GAG’) restores predicted base pairing at site 3 (versus an A–C mismatch, Fig. 2c ), resulting in a dramatic 2.5-fold increase in editing at synonymous site 2 ( Fig. 2f ). These data are consistent with previous observations [24] , which suggest that editing of site 2 is coupled to editing at site 3. In addition, ADAR enzymes prefer editing adenosines neighboured by a 3′-guanosine and a 5′-adenosine [32] . Adenosines mismatched to a cytosine are also favored [33] , suggesting that editing at site 3, an ‘ideal’ dADAR target, precedes editing at site 2, which may occur as a sequential byproduct under little or no selective pressure. A duplex containing splicing signals modulates RNA editing The highly conserved DCS sequence is predicted to generate a dsRNA structure encompassing the 5′-splice donor ( Fig. 3a ). We therefore used HR to precisely delete the DCS (24 nt) ( Fig. 3b ). In ‘DCS delete’ alleles of para , editing is reduced uniformly at all three sites compared with the LoxP control ( Fig. 3d , Supplementary Fig. S4a,b ). We considered the possibility that the wild-type DCS duplex retards splicing, directly or indirectly, thereby enhancing editing. As the ECS is within the intron, more efficient splicing in DCS delete may disfavour editing by removal of the intron. Next, we mutationally extended the DCS duplex by 9 bp (‘DCS zip’), hypothetically stabilizing the DCS duplex. The DCS zip mutation ( Fig. 3c ) resulted in substantially increased editing at all three sites ( Fig. 3d , Supplementary Fig. S4c ). Our data support in vitro experiments documenting the interplay between editing and splicing [34] . When the splicing machinery recognizes the donor site, the intron is removed and further processing, maturation and export should decrease the likelihood that dADAR recognizes the transcript due to loss of double-strandedness. Further, para transcripts with a wild-type intron or deleted for the DCS were properly spliced, whereas those from the DCS zip allele exhibited improper splicing ( Fig. 3e ). Sequencing of aberrant products in DCS zip animals revealed cryptic splice donor-site activation within constitutive exon 19 and upstream alternative exon h ( Fig. 3f ). All of these variants result in frameshift mutations and, if translated, substantially truncated channel proteins. Our observations strongly suggest that the DCS is involved in a structure that influences splicing, indirectly modulating editing levels in the central RNA duplex by influencing intron removal. We performed quantitative RT–PCR on RNA extracted from DCS zip and LoxP control animals ( Supplementary Fig. S5a ). This analysis revealed a significant decrease in full-length spliceoform in the DCS zip mutants compared with the LoxP control, while the presence of several aberrant spliceoforms was significantly increased in the mutant animals ( Supplementary Fig. S5b ). In addition, the DCS zip allele also gives rise to significantly more total para transcript than control, suggesting that transcription from the para locus is upregulated in DCS zip animals, perhaps to compensate for low levels of properly spliced para transcript and Para sodium channel protein. The para locus encodes the only action potential-generating sodium channel gene in Drosophila [14] , and excitability of the fly nervous system is highly sensitive to para dosage [35] . Animals hemi- or homozygous for temperature-sensitive (ts) para alleles, which reduce para expression, display ts-paralytic phenotypes, while null alleles of para result in unconditional lethality. Therefore, we assessed the phenotypic consequences of altered para splicing in our DCS zip mutant. Drosophila hemi- or homozygous for DCS zip show a significant ts-paralytic phenotype ( Fig. 4a , Supplementary Fig. S5c ), similar to other para ts alleles. To investigate the dosage of full-length functional para transcript originating from the DCS zip allele ( Fig. 3c ), we crossed females homozygous for the DCS zip allele to males null for endogenous para on the X chromosome, rescued by a duplication of para translocated to chromosome four. The lethality of female progeny from this cross demonstrates that the DCS zip allele is haploinsufficient. However, female siblings carrying the wild-type para duplication on chromosome four were rescued for viability ( Fig. 4b ). Interestingly, although males contain only one X chromosome, males hemizygous for the DCS zip allele are viable, likely due to the upregulation of genes on the X chromosome through the process of dosage compensation [36] . In summary, the extent of the DCS/donor-site duplex appears to modulate the degree of RNA editing. The level of editing in the central duplex can be ‘tuned’ up or down, and we propose that this is an effect modulated directly or indirectly through effects on splicing. Subtle changes predicted to strengthen the DCS duplex enhance editing at the molecular level, but do so at the cost of a substantial deleterious phenotypic consequence at the organismal level. 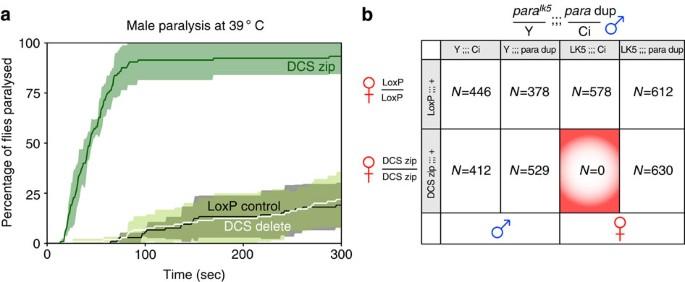Figure 4: Phenotypic consequences of aberrant splicing from the ‘DCS zip’ allele. (a) Male flies of the indicated genotypes were placed in room temperature glass vials and then submerged in a circulating 39 °C water bath. Time to first paralysis event was recorded over 5 min. Flies hemizygous for the ‘DCS zip’ allele paralyse significantly faster than those with the LoxP control allele (log-rank test;P<0.0001).N=105 flies per genotype (biological replicates). Ribbons represent s.d. (b) Virgin females homozygous for the LoxP control or ‘DCS zip’ alleles were crossed to males with aparadeletion on the X chromosome (paralk5) rescued by a wild-type chromosomal duplication on the fourth chromosome (paradup). Allele contributions from each parent are shaded. No female progeny with only one copy of the ‘DCS zip’paraallele were found (red shaded box), although this lethality is rescued by the wild-typeparaduplication on the fourth chromosome. Lethality is not observed in male progeny hemizygous for the ‘DCS zip’ allele, a phenomenon that is likely due to dosage compensation of the male X chromosome. Figure 4: Phenotypic consequences of aberrant splicing from the ‘DCS zip’ allele. ( a ) Male flies of the indicated genotypes were placed in room temperature glass vials and then submerged in a circulating 39 °C water bath. Time to first paralysis event was recorded over 5 min. Flies hemizygous for the ‘DCS zip’ allele paralyse significantly faster than those with the LoxP control allele (log-rank test; P <0.0001). N =105 flies per genotype (biological replicates). Ribbons represent s.d. ( b ) Virgin females homozygous for the LoxP control or ‘DCS zip’ alleles were crossed to males with a para deletion on the X chromosome ( para lk5 ) rescued by a wild-type chromosomal duplication on the fourth chromosome ( para dup). Allele contributions from each parent are shaded. No female progeny with only one copy of the ‘DCS zip’ para allele were found (red shaded box), although this lethality is rescued by the wild-type para duplication on the fourth chromosome. Lethality is not observed in male progeny hemizygous for the ‘DCS zip’ allele, a phenomenon that is likely due to dosage compensation of the male X chromosome. Full size image The HP structure is required for editing site selection The highly conserved intronic HP structure ( Fig. 5a ) has no obvious relationship to either the ECS or DCS duplexes, and is without precedence in other known ADAR targets. Surprisingly, deletion of the HP preferentially abolished editing at site 1 ( Fig. 5g , Supplementary Fig. S4d ). Although the nucleotide sequence of the HP stem differs between species, comparative sequence analyses revealed extensive sequence co-variation, maintaining base pairing ( Supplementary Fig. S6a,b ), suggesting that the structure ( Fig. 5b ) rather than primary sequence is necessary for editing. In particular, two unpaired bulged regions of the HP stem are almost invariably pyrimidines, and the HP stem therefore resembles a ‘barbell.’ We introduced the ‘HP zip’ mutation, which base pairs most of the bulged pyrimidines, converting the HP stem into a more perfect duplex ( Fig. 5c ). The HP zip mutation preferentially reduced editing at site 1, indicating the modulatory nature of the unpaired residues in the HP ( Fig. 5g , Supplementary Fig. S4e ). 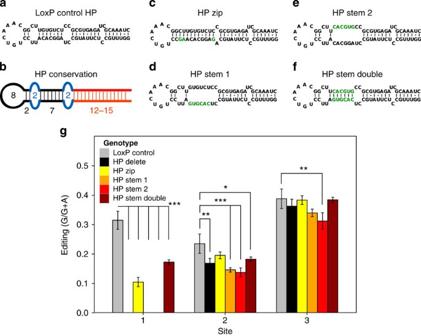Figure 5: Editing at site 1 within the central duplex requires the HP element. (a) The highly conserved predicted wild-type HP element. (b) Conservation of the HP acrossDrosophilidae. Black regions of the structure are conserved, while red are variable. Blue represents conserved pyrimidine bulges. Numbers refer to the nucleotides in the loops or base pairs in the stem. (c) The ‘HP zip’ mutation pairs some of the bulged, conserved pyrimidines (green) into the HP stem. (d) The ‘HP stem 1’ mutation introduces a destabilizingPacI site into one side of the stem, while (e) the ‘HP stem 2’ mutation introduces thePacI mutation from the opposite side. (f) Combining the HP stem 1 and 2 mutations (‘HP stem double’) restores predicted base pairing in the HP stem. (g) Deleting the HP (black) results in a selective loss of editing at site 1 compared to the LoxP control (grey), while pairing the pyrimidine bulges (‘HP zip’; yellow) results in a reduction of editing at site 1 compared with the LoxP control. Both the ‘HP stem 1’ and ‘2’ mutations (orange and red, respectively) selectively abolish editing at site 1, while the restorative double mutation (‘HP stem double’; brown) rescues editing at site 1. Bars represent 95% confidence intervals from three biological replicates (*P<0.05, **P<0.001, ***P<0.0001, one-way ANOVAs with Dunnettpost-hoctests (α=0.05), please seeSupplementary Fig. S10afor raw data and specificP-values). Figure 5: Editing at site 1 within the central duplex requires the HP element. ( a ) The highly conserved predicted wild-type HP element. ( b ) Conservation of the HP across Drosophilidae . Black regions of the structure are conserved, while red are variable. Blue represents conserved pyrimidine bulges. Numbers refer to the nucleotides in the loops or base pairs in the stem. ( c ) The ‘HP zip’ mutation pairs some of the bulged, conserved pyrimidines (green) into the HP stem. ( d ) The ‘HP stem 1’ mutation introduces a destabilizing Pac I site into one side of the stem, while ( e ) the ‘HP stem 2’ mutation introduces the Pac I mutation from the opposite side. ( f ) Combining the HP stem 1 and 2 mutations (‘HP stem double’) restores predicted base pairing in the HP stem. ( g ) Deleting the HP (black) results in a selective loss of editing at site 1 compared to the LoxP control (grey), while pairing the pyrimidine bulges (‘HP zip’; yellow) results in a reduction of editing at site 1 compared with the LoxP control. Both the ‘HP stem 1’ and ‘2’ mutations (orange and red, respectively) selectively abolish editing at site 1, while the restorative double mutation (‘HP stem double’; brown) rescues editing at site 1. Bars represent 95% confidence intervals from three biological replicates (* P <0.05, ** P <0.001, *** P <0.0001, one-way ANOVAs with Dunnett post-hoc tests ( α =0.05), please see Supplementary Fig. S10a for raw data and specific P -values). Full size image The ‘barbell’ structure of the HP is preserved in most species of Drosophilidae ( Supplementary Fig. S6a,b ). However, D. willistoni subgroup members lack the HP barbell structure ( Supplementary Fig. S6c ). We wanted to assess whether this natural variation of the HP, resembling the HP zip synthetic allele, alters editing ( Fig. 5c ). We compared editing at site 1 to editing at site 3 in species across Drosophilidae ( Supplementary Fig. S1 ). Editing at site 1 was significantly decreased in two closely related species, D. willistoni and D. equinoxialis , which lack the canonical barbell shape ( Supplementary Fig. S6c,d ). These data further suggest that the barbell shape serves to modulate editing at site 1. To test whether the HP stem sequence is necessary for editing at site 1, we introduced helix-disrupting mutations in the 5′ or 3′ side of the stem ( Figs. 5d,e ). The ‘HP stem 1’ and ‘HP stem 2’ mutations both selectively abolish editing at site 1, while combining these two compensatory mutations (‘HP stem double,’ Fig. 5f ) rescues editing at the first adenosine ( Fig. 5g , Supplementary Fig. S4f–h ). Thus, editing at site 1 requires both the presence of the HP as well as the specific paired and unpaired bases within that structure, while two other adenosines only 10 nucleotides away are unaffected by the presence and integrity of the HP. A long-range tertiary PK is mediated by the HP A closer inspection of both the HP primary sequence as well as its potential to contribute to other structural elements was revealing. First, although the HP stem covaries between Drosophila species, the HP loop is completely invariant ( Fig. 5b , Supplementary Fig. S3c ). Second, a short sequence just 3′ to the ECS is also completely conserved, is not predicted to base pair and creates a docking site for the HP loop sequence—a potential tertiary PK interaction ( Fig. 6a ). Such interactions are very difficult to predict with current RNA folding software programs. Furthermore, there is no precedence for the requirement of a long distance tertiary structural element directing specific RNA editing in a different dsRNA helix. 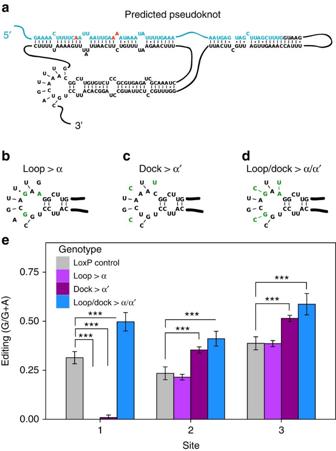Figure 6: The HP is involved in a tertiary PK that directs selective editing in the central duplex and can be functionally replaced. (a) The predicted intronic tertiary PK is composed of seven base pairs. Exon, blue; intron, black; editing sites, red. (b) The ‘Loop >α’ mutation alters three nucleotides in the HP loop (green) so that the sequence recapitulates the α sequence from the group II self-splicing intron. (c) The ‘Dock >α′’ mutation introduces three nucleotide changes (green) in the docking site of the predictedparaPK, altering the sequence into that of the self-splicing intron α′ sequence. (d) The double ‘Loop/dock>α/α′’ mutation restores the predicted PK interaction using the α and α′ sequences (green) from the group II self-splicing intron kissing-loop interaction. (e) Both the ‘Loop >α’ and the ‘Dock >α′’ mutation (light and dark purple, respectively) abolish editing at site 1, while the double mutation, ‘Loop/dock>α/α′’ (blue) rescues editing at this site compared to the LoxP control (grey). Bars represent 95% confidence intervals from three biological replicates (***P<0.0001, one-way ANOVAs with Dunnettpost-hoctests (α=0.05), please seeSupplementary Fig. S10afor raw data and specificP-values). Figure 6: The HP is involved in a tertiary PK that directs selective editing in the central duplex and can be functionally replaced. ( a ) The predicted intronic tertiary PK is composed of seven base pairs. Exon, blue; intron, black; editing sites, red. ( b ) The ‘Loop >α’ mutation alters three nucleotides in the HP loop (green) so that the sequence recapitulates the α sequence from the group II self-splicing intron. ( c ) The ‘Dock >α′’ mutation introduces three nucleotide changes (green) in the docking site of the predicted para PK, altering the sequence into that of the self-splicing intron α′ sequence. ( d ) The double ‘Loop/dock>α/α′’ mutation restores the predicted PK interaction using the α and α′ sequences (green) from the group II self-splicing intron kissing-loop interaction. ( e ) Both the ‘Loop >α’ and the ‘Dock >α′’ mutation (light and dark purple, respectively) abolish editing at site 1, while the double mutation, ‘Loop/dock>α/α′’ (blue) rescues editing at this site compared to the LoxP control (grey). Bars represent 95% confidence intervals from three biological replicates (*** P <0.0001, one-way ANOVAs with Dunnett post-hoc tests ( α =0.05), please see Supplementary Fig. S10a for raw data and specific P -values). Full size image We were struck by the similarity of the predicted para PK to a structural element of the group II self-splicing intron from an extremophilic bacterium [37] . In this autocatalytic intron, the α/α′ kissing-loop interaction scaffolds the formation of a five-way helical junction necessary for self-catalysis ( Supplementary Fig. S7 ) [38] . The primary sequence of the α/α′ kissing-loop interaction differed from that of the para HP loop/dock interaction at only three positions. We mutationally converted the HP loop sequence to the α sequence from the kissing-loop interaction ( Fig. 6b ) and the docking site into that of the α′ ( Fig. 6c ). We found that these mutations, designed to disrupt the putative tertiary PK, independently, selectively and completely abolish editing at para site 1 ( Fig. 6e , Supplementary Fig. S4i,j ). Combining the mutations in the double mutant, recapitulating the naturally occurring α/α′ kissing loop within the paralytic intron ( Fig. 6d ), restores editing ( Fig. 6e , Supplementary Fig. S4k ). Thus, our data demonstrate that the tertiary PK exists in vivo , uses a structure similar to a known example, and selectively directs the RNA-editing enzyme to deaminate only one of the three nearby edited adenosines in a separate duplex. The RNA informational complement of only four nucleotides, amplified by simple base-pairing rules, nevertheless allows for an infinite variety of secondary and tertiary structures, surfaces, and chemistries. In silico approaches, such as comparative genomics and structural predictions, are useful in identifying base pairing interactions. However, higher order RNA structures may be difficult to predict. Most structural studies of ADAR targets focus on the necessity of a central RNA duplex containing the adenosines destined for modification. In contrast, our study revealed distinct structural elements that have roles in both modulating and specifying sites of RNA editing in vivo . Many A-to-I editing sites are found near intron–exon boundaries, where edited adenosine(s) and splicing signals lie in the same dsRNA region [34] . The highly conserved DCS/donor-site RNA duplex suggests a balance between splicing and editing; postponing splicing by occlusion of splicing signals would extend time for RNA folding, ADAR binding or both, resulting in increased editing. The deletion of the DCS decreases editing overall and appears to have no deleterious effect on splicing. Thus, the DCS may serve as an editing modulator. Interestingly, the predicted DCS of Musca domestica is more extensive and a fourth adenosine is edited within this structure ( Supplementary Fig. S8a,b,e ) supporting the notion that DCS has a role in splicing and editing. It is tempting to propose that deleting the DCS exerts effects by improving the rate with which splicing signals are accessed by the spliceosome, and thus the rapidity of intron removal. However, further experiments would be necessary to determine the exact role of the DCS. We previously reported that the ‘no action potential temperature-sensitive’ ( mle napts ) mutation in the maleless dsRNA helicase results in a ‘splicing catastrophe’ [24] , causing exon skipping due to failure to utilize the 5′-donor site of exon 19, and a ts-paralytic phenotype due to lack of sufficient full-length para transcripts. The present study further shows that aberrant splicing of para and ts-paralyisis can be caused by increasing base pairing of the structure encompassing the same 5′-donor site. The DCS zip mutation adds 7 intronic nucleotides 271 nucleotides from the splice donor ( Fig. 3c ), extending the DCS/donor-site helix. Even this modest non-coding change results in a dramatic increase in RNA editing at the cost of cryptic donor-site activation ( Fig. 3f ). Owing to this aberrant splicing, we hypothesize that fewer functional sodium channel transcripts are produced ( Supplementary Fig. S5b ), decreasing channel expression. One interesting difference between this phenomenon and the effect of the mle napts mutation is that correctly spliced para transcripts in mle napts show decreased levels of RNA editing. We do not see this as being inconsistent with a splicing interaction, as the mutant Mle protein produced from mle napts was proposed to ‘stall’ on the dsRNA structure. The stalled helicase could potentially sterically interfere with ADAR binding, which would not be the case in the DCS zip allele, in which increased editing is seen. An intronic duplex distant from splicing signals in the mammalian Gabra-3 transcript was recently reported to stimulate specific editing [28] . The authors hypothesized that the duplex serves to generically increase ADAR concentration locally, differing from our proposed mechanism. Sodium channel abundance affects Drosophila behaviour, development, reproduction and aging [39] . Flies hemi- or homozygous for the DCS zip allele are ts-paralytic ( Fig. 4a , Supplementary Fig. S5c ), consistent with para alleles that confer phenotypes due to loss of para activity [14] . The substantial increase in editing in the DCS zip mutant comes at the expense of splicing defects, explaining why the DCS is not larger in size than observed. Splicing and editing occur co-transcriptionally [40] , and recent evidence points toward a role for RNA structure in splicing [41] , [42] . Our data suggest that an RNA duplex sequesters splicing signals and finely tunes RNA editing levels by directly or indirectly influencing splicing ( Fig. 7a ). A slow polymerase could also indirectly influence intron removal. Interestingly, editing levels increase in Drosophila carrying a mutant ‘slow’ RNA polymerase II compared with Canton-S wild-type animals ( Fig. 7b–c ). The C4 point mutation confers a slower elongation rate on RNA polymerase II, and affects alternative splicing of endogenous genes in both human cells and Drosophila [43] . We speculate that slower constitutive splicing (due to slowed polymerase) results in an increased level of editing. 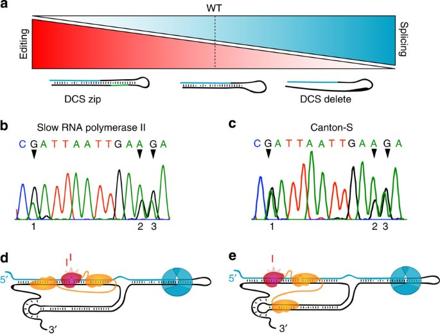Figure 7: A model forparalyticpre-mRNA editing and splicing. (a) Editing (red) and splicing (blue) are inversely correlated. When splicing is very slow or inefficient, editing is high, for example, in thepara‘DCS zip’ allele. If splicing is rapid or highly efficient, theparalyticstructure is quickly resolved, resulting in lower levels of editing, for example, transcripts from thepara‘DCS delete’ allele. (b) Editing in the ‘slow’ RNA polymerase II mutant fly is higher at all three sites than in Canton-S (c). (d) dADAR dsRNA-binding domains (orange) bind to only the ECS to edit sites 2 and 3 into inosine (red). This occurs before the splicing machinery (blue) recognizes the splice donor. (e) dADAR binds to the ECS and HP duplexes to correctly position the catalytic domain (red) to editparasite 1. Figure 7: A model for paralytic pre-mRNA editing and splicing. ( a ) Editing (red) and splicing (blue) are inversely correlated. When splicing is very slow or inefficient, editing is high, for example, in the para ‘DCS zip’ allele. If splicing is rapid or highly efficient, the paralytic structure is quickly resolved, resulting in lower levels of editing, for example, transcripts from the para ‘DCS delete’ allele. ( b ) Editing in the ‘slow’ RNA polymerase II mutant fly is higher at all three sites than in Canton-S ( c ). ( d ) dADAR dsRNA-binding domains (orange) bind to only the ECS to edit sites 2 and 3 into inosine (red). This occurs before the splicing machinery (blue) recognizes the splice donor. ( e ) dADAR binds to the ECS and HP duplexes to correctly position the catalytic domain (red) to edit para site 1. Full size image The physiological importance of RNA editing on Para protein function is unknown, although editing occurs near sites implicated in human SCN1A-based epilepsy. Nevertheless, we assayed behavioural phenotypes in mutants that encode the extremes of editing: the GAG mutant (fully edited), resulting in Para channels with Arg and Asp residues inserted, and the ECS delete mutant (fully unedited), resulting in genomically encoded Glu and Asn residues. These two mutations conferred no detectable locomotor, diurnal or mating behavioural phenotypes ( Supplementary Fig. S9 ). We conclude that RNA editing at these sites results in subtle alterations in channel function and behaviour that are too subtle for our methods of detection. Complex tertiary interactions that extend base pairing to extrahelical and non-canonical base pairs in dsRNA structures are frequently essential to function, and are exemplified by the PK. For example, protein synthesis relies on a central PK in 30S ribosomal RNA to scaffold three major structural domains [44] . Likewise, telomerase depends on a core PK within its RNA component [45] . PKs also figure prominently in viral mRNAs during the process of ribosomal frameshifting [46] . The PK interaction we report here is unique in directing specific RNA editing. Length and helix discontinuities (loops and bulges) within central RNA duplexes are usually thought to limit ADAR activity to specific adenosines [47] . We propose that the exon/ECS duplex is inconsistent in either size or structure with a standard binding of dADAR to the duplex for editing at site 1, and necessitated the evolution of a more complex structure to orchestrate binding of dADAR for site 1 editing ( Fig. 7d,e ). M. domestica and Sarcophaga bullata show RNA editing at sites 1–3 ( Supplementary Fig. S8a,d ), and comparative genomics reveal a conserved HP, located between DCS and ECS elements, with an invariant eight-nucleotide loop ( Supplementary Fig. S8a–c ). Curiously, the loop sequence differs from that seen in Drosophilidae , and no obvious conserved docking site was detected. The paralytic PK interaction reported herein encompasses seven Watson–Crick base-pairing interactions. Although the HP loop and docking site are absolutely conserved in all studied Drosophilidae species ( Fig. 5b , Supplementary Fig. S3c ), replacing PK sequences with a naturally occurring motif supported editing ( Fig. 6e ). The kissing-loop interaction in the group II intron and the para HP loop/docking site interaction share 5/8-nucleotide identity, raising the question of whether there may be a constraint on this tertiary structural motif. Although the Drosophila para PK sequences are invariant, the α/α′ sequences from group II introns do co-vary [48] . Indeed, seven base pairs is thought to be a minimum required for rapid nucleotide annealing [49] , although certain kissing loops comprising as little as two base pairs can have surprising stability [50] . Another persistent question is whether this novel structural arrangement is subject to novel regulatory inputs, especially from the environment. For example, might this type of site be sensitive to temperature, cellular stress or even function to sense metabolites in a manner similar to a riboswitch? Recent effort in the editing field has focused on identification of new editing sites via RNAseq, thereby compiling comprehensive ‘inosinomes’ [51] . Yet these studies are often controversial [52] , and pose substantial analytical challenges due to false positives [53] . Editing is implicated in an expanding list of diseases, including breast cancer [54] , suicidal depression [55] and amyotrophic lateral sclerosis (ALS). Substantial evidence points toward ADAR2 mis-regulation in motor neurons of ALS patients [56] , and recent identification of a hexanucleotide repeat associated with ALS [57] has strengthened the hypothesis that aberrant RNA processing is involved in ALS, possibly through the sequestration of RNA-binding proteins, such as ADAR, with irregular transcripts in inclusion bodies [58] . Broadly, our observations suggest that proximity of editing sites does not imply functional coupling. Future efforts to find polymorphisms affecting editing levels need not assume that canonical ECS elements are sufficient to determine editing extent and specificity. Lastly, our data on complex tertiary interactions could assist in the design of artificial editing substrates, enabling the co-option of endogenous ADAR enzymes as tools in specific RNA therapies. For example, a 937-bp antisense sequence designed to trigger RNA editing and degradation of the HIV env transcript, is already in clinical trials [59] . Further, the adenosine preference of the human ADAR protein is mutable [19] , and the enzyme itself therefore presents a possible target for genetic disease therapy. Sequence alignments Sequence alignments were performed using the ClustalW multiple sequence alignment package included with MacVector tm 7.2 (Accelrys Inc.). Open and extend gap penalties were set to 1.0. The 37 species alignment was then used for the cladogram in the Supplementary material . The cladogram was generated using the neighbor-joining method, bootstrap (1,000 reps). RNA structural predictions Structural predictions for regions encompassing all elements and the HP element alone were performed using the SFOLD web-based algorithm ( http://sfold.wadsworth.org/cgi-bin/index.pl ) using the SRNA package to generate general features and output for statistical RNA folding. Drosophila stocks Stocks were maintained at 25 °C under 12-h light/dark cycles on standard cornmeal molasses food. The ‘slow’ RNA polymerase mutant Drosophila line ‘RpII215 C4 ’ was obtained from Bloomington Stock Center (no. 3663). Y.A. Savva and J.E.C. Jepson provided the dADAR hyp and dADAR 5G1 Drosophila lines B. Ganetzky supplied the para lk5 ;;;para dup/Ci stock. Ends-out HR of the paralytic locus We performed ends-out HR after Staber et al. [31] . This technique involves two 2.5 Kb arms homologous to the para locus and flanked by recognition sites for the Flp and I-Sce I endonucleases. We cloned and sequenced two homology arms in pTOPO (Life Technologies) and then ligated them into a p[w25.2] targeting vector. Primers used for Arm 1 were: PTMARM1-F, 5′-TCGTACGCTGTTGCCGAGTAGTGGAATCATCTTAG-3′; PTMARM1-R, 5′-TGGCGCGCCAGAGCGGAGCAAGAAATTCCATCGG-3′ Primers used for Arm 2 were: PTMARM2-F, 5′-TGGTACCGAGAAGATACTATGTATTTTGGTAGC-3′; PTMARM2-R, 5′-TGCGGCCGCGACCAATCGTGTTGCATGTATGGTTCC-3′ We achieved mutations in the desired region using the Quik Change II XL Site-directed Mutagenesis Kit (Agilent Technologies). The mini-gene white + , situated between the arms and flanked by LoxP sites, acts as a selectable eye colour marker and is removed later with Cre-recombinase. The vector was introduced into the Drosophila genome by injection (Genetic Services, Inc.). We targeted the endogenous para locus so as to generate multiple independent events. We removed the white + marker from each line by crossing in Cre-recombinase and isolating individuals carrying targeted alleles with a single LoxP remnant. We then validated targeted alleles via Sanger sequencing (University of Wisconsin Biotechnology Center). RNA-editing analyses For each mutation analysed we performed six analyses, two PCRs each from three independent Drosophila HR lines. Species-specific editing data were obtained from three PCR replicates derived from a single RNA sample. For each sample, we extracted RNA from male heads ( N =15–20) using Tri Reagent (Molecular Research Center, Inc.). We amplified cDNAs via RT–PCR using a para -specific primer ( Supplementary Table S1 ), performed PCR and electrophoresed samples on agarose gels. Species-specific editing data were obtained by designing PCR and RT primers to regions of homologous sequence ( Supplementary Table S1 ). We cleaned the products using Wizard Gel and PCR Cleanup Kits (Promega) and detected editing by Sanger sequencing (University of Wisconsin Biotechnology Center) using a site-specific primer ( Supplementary Table S1 ). We determined editing ratios by measuring the area under select A and G nucleotide traces in Adobe Photoshop. Identification of cryptic splice site activation We cleaned PCR products, as above, and sequenced individual products. Temperature-sensitivity paralysis assay We raised Drosophila at room temperature (18 °C) and tested all animals within 24 h after ecclosion. We mouth pipetted single flies into room temperature glass vials, which we then submerged in a circulating 39 °C water bath. We measured time from submersion until first detectable paralytic event, defined as 5 s lying on the back or (rarely) side. We tested 105 flies per genotype (35 each from three independent HR lines) per sex. Quantitative RT–PCR assay We isolated mRNA from 40 male Drosophila heads per biological replicate using oligo d(T) 25 magnetic beads (New England BioLabs). We normalized and reverse-transcribed the mRNA using the iScript cDNA Synthesis Kit (Bio-Rad). We then performed quantitative RT–PCR using the SYBR Green PCR Master Mix (Applied Biosystems) and ran plates on the 7500 Fast Real-Time PCR System machine (Applied Biosystems). We performed three technical replicates per biological replicate, and three biological replicates for both the LoxP control and DCS zip lines. We used primers specific to the mature GAPDH transcript to normalize the data from replicates ( Supplementary Table S1 ). To detect total para transcript, we designed primers specific to the 3′ most exon–exon junction of the mature para mRNA. To detect spliceoforms, we designed primer pairs within exons 19 and 20 (see Supplementary Fig. S5a , Supplementary Table S1 ). We performed melting curves on each PCR product to ensure primer specificity. Activity analysis Multiple lines of HR-constructed flies were first backcrossed to Canton-S for five generations. Three lines of each genotype were used in subsequent behavioural assays. Total activity was measured using individual activity monitors (TriKinetics). Each monitor consists of a horizontal glass capillary bisected by an infrared beam. Activity is quantified as the total number of beam breaks in 30-min bins over a 24-h period. Flies of the indicated genotypes were raised in 12-h/12-h light/dark conditions. Individual male flies (3–5 days post-eclosion) were placed in monitors and allowed to acclimate for 12 h before data collection. Data were collected and averaged over 3 days. Mating analysis Mating analyses were conducted between 0700 and 0900 hours, by a single observer blind to male genotype. Virgin males of the indicated genotypes and Canton-S virgin females were isolated in un-yeasted vials and aged 4 days. During each assay, the male was acclimated to the mating chamber for 5 min before the female was added. All assays were conducted for 10 min or until successful copulation. Latency is defined as time before male orientation. Time spent courting is the proportion of the total assay time that the male spent following, singing, dancing, tapping and licking the female. Courting time before copulation is defined as the total time from the start of the assay until copulation by successful males. Statistical analyses For editing analyses, we performed one-way ANOVAs ( α =0.05) followed by Dunnett post-hoc tests. * P <0.05, ** P <0.001, *** P <0.0001. All experimental lines were compared to LoxP control lines. For specific P- values please see Supplementary Fig. S9 . For paralysis analyses, we performed log-rank tests on the raw data. We performed one-way ANOVAs on qRT–PCR data after Rieu and Powers [60] . How to cite this article: Rieder, L. E. et al. Tertiary structural elements determine the extent and specificity of messenger RNA editing. Nat. Commun. 4:2232 doi: 10.1038/ncomms3232 (2013).